Neurofilament sidearms modulate parallel and crossed-filament orientations inducing nematic to isotropic and re-entrant birefringent hydrogels Neurofilaments are intermediate filaments assembled from the subunits neurofilament-low, neurofilament-medium and neurofilament-high. In axons, parallel neurofilaments form a nematic liquid-crystal hydrogel with network structure arising from interactions between the neurofilaments’ C-terminal sidearms. Here we report, using small-angle X-ray-scattering, polarized-microscopy and rheometry, that with decreasing ionic strength, neurofilament-low–high, neurofilament-low–medium and neurofilament-low–medium–high hydrogels transition from the nematic hydrogel to an isotropic hydrogel (with random, crossed-filament orientation) and to an unexpected new re-entrant liquid-crystal hydrogel with parallel filaments—the bluish-opaque hydrogel—with notable mechanical and water retention properties reminiscent of crosslinked hydrogels. Significantly, the isotropic gel phase stability is sidearm-dependent: neurofilament-low–high hydrogels exhibit a wide ionic strength range, neurofilament-low–medium hydrogels a narrow ionic strength range, whereas neurofilament-low hydrogels lack the isotropic gel phase. This suggests a dominant regulatory role for neurofilament-high sidearms in filament reorientation plasticity, facilitating organelle transport in axons. Neurofilament-inspired biomimetic hydrogels should therefore exhibit remarkable structure-dependent moduli and slow and fast water-release properties. Neurofilaments (NFs) are type IV intermediate filaments [1] , [2] , [3] , [4] unique to neuronal cells, where their physiologically relevant state in axons is a space-filling nematic liquid-crystal (LC) hydrogel (with parallel filament orientation) stabilizing the axonal calibre and protecting against mechanical stress [1] , [5] , [6] , [7] . The NF network, which acts as a scaffold for microtubules, must be sufficiently flexible to allow for the transport of relatively large organelles (typically larger than the interfilament spacings) trafficking along microtubules immersed within the network [8] , [9] , [10] , [11] . NFs comprise three distinct subunits—NF-Low (NF-L), NF-Medium (NF-M), and NF-High (NF-H)—with similar design elements consisting of an unstructured N-terminal tail, an alpha-helical core and an unstructured C-terminal sidearm ( Fig. 1a ) [1] , [2] , [3] , [4] . The NF subunits form the coiled-coil dimers neurofilament-low–low (NF-LL), neurofilament-low–medium (NF-LM) and neurofilament-low–high (NF-LH) stabilized by the alpha-helical cores, which further assemble to form the flexible, 10 nm diameter NF filament with radially protruding unstructured C-terminal sidearms ( Fig. 1b ), the building block of the NF network. The sidearms, with varying length and charge distribution, are responsible for imparting distinct functions to NF networks, many of which remain to be elucidated. In mature neurons, the composition of the NF subunits is regulated over a narrow range (for example, in mouse the mole fraction is 7:3:2 for NF-L:NF-M:NF-H) with incorrect compositions or subunit phosphorylation resulting in the disruption of the NF network due to aberrant sidearm interactions or NF subunit over-accumulation. Motor neuron diseases including amyotrophic lateral sclerosis (Lou Gehrig’s disease) show evidence of such disrupted NF networks [12] , [13] , [14] . 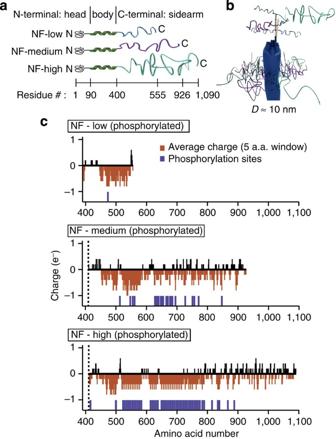Figure 1: Neurofilament assembly and charge distributions. (a) Schematic depicting the unifying tripartite structure of NF-L, NF-M and NF-H subunits: the helical body is flanked by two unstructured domains, the N-terminal head and the C-terminal sidearms. (b) NFs are assembled from dimers of the subunits, where NF-L is a necessary component of dimers. Parallel dimers (NF-LL, NF-LM and NF-LH) assemble into antiparallel half-staggered tetramers that further assemble into octomeric protofilaments. Four protofilaments form the mature 10 nm filament. (c) C-terminal sidearm charge as a function of the amino acid residues (averaged over five residues; sequences and phosphorylation sites, reported as purple bars below the sidearms, are from the NCBI protein database) for NF-L, NF-M and NF-H (pH 6.8). For NF-L (P02548.3) and NF-M (O77788.3), bovine sequences were used. Mouse sequence was used for NF-H (NP_035034.2). The 158-residue NF-L sidearm (net charge ≈−40e) has a nearly contiguous negative domain over ≈2/3 of its length, with cationic residues near the filament body and tip of the C-terminus. For NF-M and NF-H the net charge and charge distribution of sidearms is dependent on the degree of phosphorylation. The NF-M and NF-H sidearms have 22 and 48 potentially phosphorylated serine residues, respectively16,17,18. The net charge of unphosphorylated 514-residue NF-M sidearm increases from ≈−46e to ≈−90e upon phosphorylation (seeSupplementary Fig. S1) with negative regions along most of the sidearm and cationic residues near the filament body and distributed from the central region towards the C-terminus. The 679-residue NF-H sidearm is weakly charged (≈−7e) before phosphorylation (seeSupplementary Fig. S1). Upon phosphorylation NF-H sidearm has a net charge of ≈−93e concentrated in the first half of the sidearm (with interspersed positive residues) followed by a segment of alternating positive/negative residues (790–1090) extending to the C-terminus with small net charge ≈−6e. NF-M has a smaller alternating positive/negative region (residues 849–926, ≈−3e net charge) near the C-terminus. Figure 1: Neurofilament assembly and charge distributions. ( a ) Schematic depicting the unifying tripartite structure of NF-L, NF-M and NF-H subunits: the helical body is flanked by two unstructured domains, the N-terminal head and the C-terminal sidearms. ( b ) NFs are assembled from dimers of the subunits, where NF-L is a necessary component of dimers. Parallel dimers (NF-LL, NF-LM and NF-LH) assemble into antiparallel half-staggered tetramers that further assemble into octomeric protofilaments. Four protofilaments form the mature 10 nm filament. ( c ) C-terminal sidearm charge as a function of the amino acid residues (averaged over five residues; sequences and phosphorylation sites, reported as purple bars below the sidearms, are from the NCBI protein database) for NF-L, NF-M and NF-H (pH 6.8). For NF-L (P02548.3) and NF-M (O77788.3), bovine sequences were used. Mouse sequence was used for NF-H (NP_035034.2). The 158-residue NF-L sidearm (net charge ≈−40e) has a nearly contiguous negative domain over ≈2/3 of its length, with cationic residues near the filament body and tip of the C-terminus. For NF-M and NF-H the net charge and charge distribution of sidearms is dependent on the degree of phosphorylation. The NF-M and NF-H sidearms have 22 and 48 potentially phosphorylated serine residues, respectively [16] , [17] , [18] . The net charge of unphosphorylated 514-residue NF-M sidearm increases from ≈−46e to ≈−90e upon phosphorylation (see Supplementary Fig. S1 ) with negative regions along most of the sidearm and cationic residues near the filament body and distributed from the central region towards the C-terminus. The 679-residue NF-H sidearm is weakly charged (≈−7e) before phosphorylation (see Supplementary Fig. S1 ). Upon phosphorylation NF-H sidearm has a net charge of ≈−93e concentrated in the first half of the sidearm (with interspersed positive residues) followed by a segment of alternating positive/negative residues (790–1090) extending to the C-terminus with small net charge ≈−6e. NF-M has a smaller alternating positive/negative region (residues 849–926, ≈−3e net charge) near the C-terminus. Full size image The NF sidearms are polyampholytes (containing both positively and negatively charged amino acids) with a net negative charge ( Fig. 1c and Supplementary Fig. S1 for more details) [15] , [16] , [17] , [18] . The presence of oppositely charged residues allows for the possibility of interfilament interactions through the formation of favourable ionic bonds between interpenetrating sidearms leading to large-scale network formation [19] , [20] , [21] . Recent small-angle-X-ray-scattering (SAXS) experiments of nematic LC-NF hydrogels (labelled N G ) have clarified the role of the three sidearms in determining interfilament spacings mimicking conditions in dendrites (consisting of NF-LM nematic hydrogels with little or no NF-H component) and axons (consisting of NF-LMH nematic hydrogels) [22] . Furthermore, SAXS osmotic pressure studies of N G hydrogels have described a transition to a highly condensed gel network at high pressures, which is a direct signature of the onset of short-range attractive ionic bonds between antiparallel sidearms [23] . The current study was designed to alter the interfilament electrostatic interactions through variations of ionic strength ( C S , which included (1:1) NaOH and KCl salts), in order to understand the role of the polyampholyte sidearms in driving the formation of different NF hydrogel phases, with distinct underlying network structure, filament orientation and mechanical properties. Modulating the electrostatic interactions through changes in salt concentration in binary (NF-LL, NF-LM and NF-LH) and ternary (NF-LMH) systems, in vitro , closely mimics such modulations, in vivo , through subunit phosphorylation or dephosphorylation (see Supplementary Fig. S1 ) at near-constant salinity. Purified and reassembled 10 nm NFs form networks, which with decreasing ionic strength, transition from the anisotropic nematic LC hydrogel (N G , with parallel filament orientation) to an isotropic hydrogel (I G , with random, crossed-filament orientation) and to an unexpected new re-entrant anisotropic LC hydrogel (a bluish-opaque hydrogel, B G , with parallel filament orientation). We find that the NF-LH hydrogels exhibit a wide range of stability for the I G phase (Δ C S ≈70 mM), NF-LM hydrogels a narrow range (Δ C S ≈10 mM), and NF-Low hydrogels lack the I G phase entirely. This remarkable sidearm dependence for the isotropic I G phase stability suggests a dominant regulatory role for NF-H sidearms in filament re-orientation plasticity. The data suggest a model where, at low C S , the B G phase is stabilized by zipped short-range ionic bonds between unstructured polyampholyte sidearms. Unzipping of weaker ionic bonds, at intermediate C S , drives the transition to the I G phase where random, crossed-filament orientation lowers the longer-ranged electrostatic repulsions due to net-negatively charged sidearms. At even higher C S , screening of repulsions drives the transition to an Onsager-type N G phase. The isotropic and LC hydrogels, with reversible transitions between them, are found to have distinct, and at very low ionic strength, very large elastic moduli reminiscent of crosslinked hydrogels. A further remarkable finding is that unlike the isotropic hydrogel, LC hydrogels (in particular, the B G phase) exhibit new functionality in their ability to retain water over very long times due to their underlying anisotropic microscopic structures. Optical characterization of NF hydrogel phase behaviour The phase behaviour of the hydrogels of different subunit composition and over a wide range of salt concentrations was mapped out using polarized optical microscopy (POM), which distinguishes between anisotropic birefringent and isotropic hydrogels arising from the underlying filament orientation. The hydrogels were prepared at the desired subunit composition and allowed to swell to their final volume in excess buffer at different monovalent salt concentrations. All hydrogels were very dilute containing between ≈1 wt% and ≈2 wt% protein reflecting the highly charged nature of the NFs (see Methods; Supplementary Tables S1–S4 ). The binary (NF-LM and NF-LH) and ternary (NF-LMH) hydrogels exhibited three distinct phases. Exemplary optical micrographs for NF-LM (70:30 wt%) hydrogels are shown in Fig. 2a,b . At high C S POM shows the existence of the previously studied nematic hydrogel with thread-like LC defect patterns indicative of long-range parallel filament orientation ( Fig. 2a ; C S =150 mM; labelled N G ) [22] . With decreasing C S the N G hydrogel transitions into an I G gel phase at intermediate C S showing complete light extinction in POM indicative of random crossed-filament orientation ( Fig. 2a ; C S =40 mM; labelled I G ). 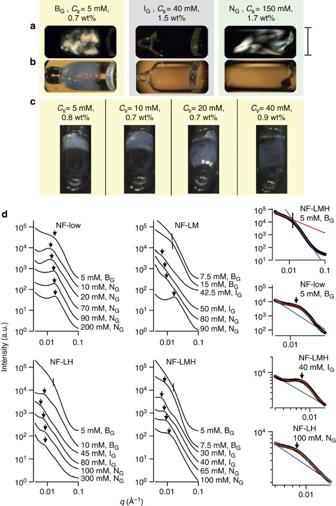Figure 2: Optical microscopy and SAXS of NF hydrogel phases. (a) Polarized optical microscopy images ( × 5 magnification) of hydrogels of copolymer NF-LM 70:30 wt% (≈3.9:1 mol:mol) in each of the three distinct monovalent-salt-induced phases: bluish-opaque gel (BG) at 5 mM, isotropic gel (IG) at 40 mM and nematic gel (NG) at 150 mM salt. For NF-LM 70:30 wt%, the BG–IGand IG–NGtransitions occur at ionic strengthCS=37.5 mM andCS=50 mM, respectively. Scale bar ≈1.5 mm. (b) Bright-field images of the same samples in (a) that reveal the partial opacity/bluish colour of BGhydrogels in contrast to the transparent IGand NGhydrogels. (c) Bright-field images of equilibrated hydrogels of copolymer NF-LM 60:40 wt% (≈2.5:1 mol:mol) that display the fading of the bluish tint in the BGhydrogel with increase in monovalent salt concentration. The images (rotated by 90° compared to (a) and (b)) show hydrogels in the same type of capillaries as seen in (b) and at the same magnification. (d) (left and middle) Exemplary SAXS profiles for hydrogels of NF-L and copolymers NF-LM 60:40 wt% (≈2.5:1 mol ratio), NF-LH 70:30 wt% (≈4.6:1 mol ratio) and NF-LMH 44:31:25 wt% (≈7:3:2 mol ratio) at different salt concentrations. Arrows and lines correspond to positions inqwhere either a correlation peak is evident (arrows) or, in some BGsamples, where the enhanced SAXS masks the correlation peak, a shoulder (marked by lines; as described in the text). A peak at higherqappears in some traces, which is due to NF form factor as it always occurs in the same position and is salt-independent. (right) Examples of fits to the correlation peaks in each of the hydrogel phases (NG, IGand BG) and a BGphase where the correlation peak is replaced by a shoulder (top profile, position determined by the intersection of tangent lines log–log plots). In addition to the (1:1) salt concentration labelled in the figures, all samples included 1 mM MgCl2. Figure 2: Optical microscopy and SAXS of NF hydrogel phases. ( a ) Polarized optical microscopy images ( × 5 magnification) of hydrogels of copolymer NF-LM 70:30 wt% (≈3.9:1 mol:mol) in each of the three distinct monovalent-salt-induced phases: bluish-opaque gel (B G ) at 5 mM, isotropic gel (I G ) at 40 mM and nematic gel (N G ) at 150 mM salt. For NF-LM 70:30 wt%, the B G –I G and I G –N G transitions occur at ionic strength C S =37.5 mM and C S =50 mM, respectively. Scale bar ≈1.5 mm. ( b ) Bright-field images of the same samples in ( a ) that reveal the partial opacity/bluish colour of B G hydrogels in contrast to the transparent I G and N G hydrogels. ( c ) Bright-field images of equilibrated hydrogels of copolymer NF-LM 60:40 wt% (≈2.5:1 mol:mol) that display the fading of the bluish tint in the B G hydrogel with increase in monovalent salt concentration. The images (rotated by 90° compared to ( a ) and ( b )) show hydrogels in the same type of capillaries as seen in ( b ) and at the same magnification. ( d ) (left and middle) Exemplary SAXS profiles for hydrogels of NF-L and copolymers NF-LM 60:40 wt% (≈2.5:1 mol ratio), NF-LH 70:30 wt% (≈4.6:1 mol ratio) and NF-LMH 44:31:25 wt% (≈7:3:2 mol ratio) at different salt concentrations. Arrows and lines correspond to positions in q where either a correlation peak is evident (arrows) or, in some B G samples, where the enhanced SAXS masks the correlation peak, a shoulder (marked by lines; as described in the text). A peak at higher q appears in some traces, which is due to NF form factor as it always occurs in the same position and is salt-independent. (right) Examples of fits to the correlation peaks in each of the hydrogel phases (N G , I G and B G ) and a B G phase where the correlation peak is replaced by a shoulder (top profile, position determined by the intersection of tangent lines log–log plots). In addition to the (1:1) salt concentration labelled in the figures, all samples included 1 mM MgCl 2 . Full size image Remarkably, with further decrease in C S the hydrogel re-enters into an anisotropic LC phase showing strong birefringence in POM with the LC texture indicative of smaller oriented NF domains compared to the high salt nematic hydrogel ( Fig. 2a ; C S =5 mM; labelled B G ). A distinguishing feature of this anisotropic phase (with parallel filament orientation) seen in bright-field optical microscopy is the partial opacity of the phase with a distinct bluish tint ( Fig. 2b , labelled B G for blue gel). The opacity/bluish tint of the B G hydrogel decreases gradually with increasing C S ( Fig. 2c , left to right panels), vanishing at the transition to the I G phase ( Fig. 2b ) with the hydrogel remaining transparent in the N G phase ( Fig. 2b ). The optical images of the B G phase show no evidence of coexistence of two phases (that is, the hydrogel is a single phase at the macroscopic level) and the origin of the bluish cloudiness—indicative of a spatially heterogeneous microstructure—is most likely microphase separation of submicron domains of high- and low-concentration NFs (discussed in more detail later). Unlike the relatively smooth surfaces at the gel–sol interface for the I G and N G phases, the B G hydrogels have a rough surface texture. In contrast to heteropolymer NF hydrogels, the NF-L hydrogels (same as NF-LL hydrogels) bypass the I G phase and transition directly from the N G to B G phase with decreasing C S . SAXS characterization of NF hydrogels SAXS was used to characterize the microstructure in the distinct hydrogel phases. The left and middle columns in Figure 2d show typical SAXS profiles for NF-L, NF-LM and NF-LMH hydrogels with decreasing C S (bottom to top) in different hydrogel phases. As described previously [22] , [23] the broad correlation peaks in the SAXS data allow us to measure the average interfilament spacing ( d=2 π /q NF ) from the peak position ( q NF ) of the maximum in the correlation peak in q -space (see Methods). A noticeable feature is the onset of enhanced SAXS for q <0.01 Å −1 in the B G phase, whereby the interfilament correlation peaks (marked by arrows in Fig. 2d and Supplementary Fig. S2 ) become less discernible. Figure 2d shows examples of fits to correlation peaks for N G , I G and B G phases (bottom to top, NF-LM, NF-LMH and NF-Low). For some of the B G hydrogels the SAXS profiles instead show a shoulder at q SH (that is, marked by lines in Fig. 2d and Supplementary Fig. S2 at the intersection of two tangent lines in a log–log plot; see for example, NF-LMH, 5 mM, Fig. 2d ). The observation of a shoulder in some B G hydrogels rather than an inflection point (indicative of a correlation peak) is most likely due to the enhanced SAXS, which increases deeper in the blue phase. The enhanced SAXS for q <0.01 Å −1 (length scales ≈62.8 nm and larger) and the presence of a shoulder at a larger q SH indicates that the B G phase heterogeneity (which is present on the scale of visible light due to the partially opaque light scattering) is present even on smaller scales. This would lead to a distribution of interfilament spacings, which, depending on the degree of heterogeneity broadens and weakens the correlation peak, or typically, with decreasing salt concentrations in the B G phase, masks it entirely (for example, in Supplementary Fig. S2 compare NF-LH 10 mM to 5 mM; NF-LMH 7.5 mM to 5 mM), giving rise to a shoulder at a length scale l SH ≈2π/q SH comparable to the average interfilament spacing found in B G samples, which show a measurable correlation peak. 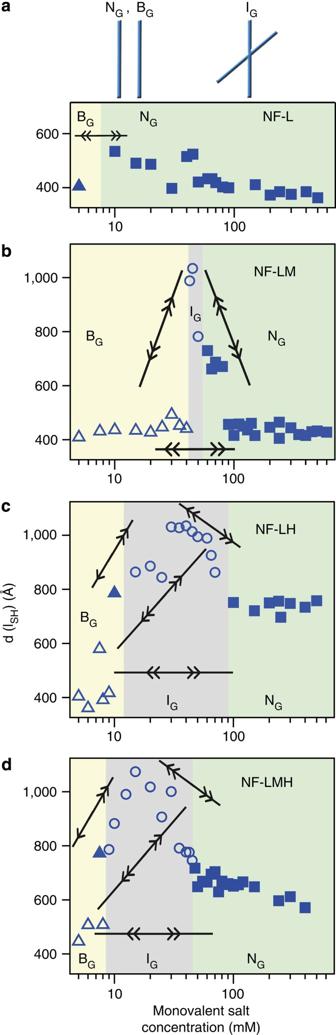Figure 3: Phase diagrams of NF hydrogels. (top) Schematics of parallel (for nematic (NG), bluish-opaque (BG) hydrogels) and crossed (for isotropic (IG) hydrogel) filament orientation. (a–d) Phase diagrams of NF-L (a), NF-LM 60:40 wt% (≈2.5:1 mol ratio) (b), NF-LH 70:30 wt% (≈4.6:1 mol ratio) (c) and NF-LMH 44:31:25 wt% (≈7:3:2 mol ratio) (d) hydrogels as a function of salt concentration. Theyaxis plots either the average interfilament spacing in each phase (d, filled squares, open circles and filled triangles for NG, IGand BGphases, respectively) or a length scalelSH=2π/qSH(open triangles in the BGphase) reflective of the inherent heterogeneity/disorder in interfilament spacings as described in the text. The BG-to-IGand IG-to-NGtransitions occur at ionic strengthCS=41±1.5 mM and 55±5 mM; 12.5±2.5 mM and 90±10 mM; and 8.5±0.5 mM and 46±1.5 mM for NF-LM, NF-LH, and NF-LMH, respectively. The homopolymer hydrogel NF-L transitions from BG-to-NGatCS=7.5±2.5 mM. The arrows indicate reversibility in transitioning between hydrogel phases. Double arrow heads imply immediate (on the order of seconds), single arrow head implies on the order of minutes. All hydrogel samples included 1 mM MgCl2in addition to the (1:1) salt concentration reported along thexaxis. Figure 3 is a composite of the POM and SAXS results (from Fig. 2 ) and shows the hydrogel phase diagrams (phases and phase boundaries from POM) with the average interfilament spacings ( d ) in each hydrogel phase (from SAXS) plotted versus C S . The data points shown in the B G phase correspond either to d-spacings from SAXS profiles showing a correlation peak (filled triangles) or to the length scale l SH =2 π /q SH (open triangles) associated with the shoulder visible in SAXS and reflective of large heterogeneity in interfilament spacings ( vide supra ). Except for the NF-L hydrogel, which lacks the isotropic phase ( Fig. 3a ), the I G phase in the NF hydrogels containing the longer NF-M and NF-H sidearms ( Fig. 3b–d ) have a larger d (that is, smaller q NF in SAXS profiles, Fig. 2d ), reflecting the larger mesh size of the isotropic network with crossed filaments, compared to the distance between parallel filaments in the N G and B G phases. To ensure that the observed hydrogel phases (B G , I G and N G ) were equilibrium states (rather than trapped states that are route-dependent), buffer exchange experiments (post-hydrogel assembly) were conducted to ensure reversibility (see Methods). The phase changes were either immediate ( Fig. 3a–d , double arrow-heads) or took a few minutes ( Fig. 3c,d , single arrow-head from I G to B G near transition) after buffer exchange. Figure 3: Phase diagrams of NF hydrogels. (top) Schematics of parallel (for nematic (N G ), bluish-opaque (B G ) hydrogels) and crossed (for isotropic (I G ) hydrogel) filament orientation. ( a – d ) Phase diagrams of NF-L ( a ), NF-LM 60:40 wt% (≈2.5:1 mol ratio) ( b ), NF-LH 70:30 wt% (≈4.6:1 mol ratio) ( c ) and NF-LMH 44:31:25 wt% (≈7:3:2 mol ratio) ( d ) hydrogels as a function of salt concentration. The y axis plots either the average interfilament spacing in each phase ( d , filled squares, open circles and filled triangles for N G , I G and B G phases, respectively) or a length scale l SH =2 π /q SH (open triangles in the B G phase) reflective of the inherent heterogeneity/disorder in interfilament spacings as described in the text. The B G -to-I G and I G -to-N G transitions occur at ionic strength C S =41±1.5 mM and 55±5 mM; 12.5±2.5 mM and 90±10 mM; and 8.5±0.5 mM and 46±1.5 mM for NF-LM, NF-LH, and NF-LMH, respectively. The homopolymer hydrogel NF-L transitions from B G -to-N G at C S =7.5±2.5 mM. The arrows indicate reversibility in transitioning between hydrogel phases. Double arrow heads imply immediate (on the order of seconds), single arrow head implies on the order of minutes. All hydrogel samples included 1 mM MgCl 2 in addition to the (1:1) salt concentration reported along the x axis. Full size image What is most striking is that although NF-LM hydrogels ( Fig. 3b ) exhibit the isotropic phase over a relatively narrow salt window (Δ C S ≈10 mM), NF-LH hydrogels ( Fig. 3c ) extend the isotropic phase over a much wider range (Δ C S ≈70 mM) to both higher and lower salt concentrations. The ternary NF-LMH hydrogel ( Fig. 3d ) shows revealing behaviour. Comparing it to NF-LM hydrogels shows that the addition of the NF-H subunit extends the I G phase primarily by suppressing the onset of the B G phase to lower C S (from ≈41.5±1.5 mM to 8.5±0.5 mM) while the I G -to-N G transition is less affected (from ≈55±5 mM to ≈46±1.5 mM) and controlled mainly by the NF-M subunit in ternary hydrogels. Similarly, comparing NF-LH to NF-LMH gels shows that the addition of NF-M suppresses the I G phase by extending the N G phase to lower C S (from ≈90±10 mM to ≈46±1.5 mM) while the I G -to-B G transition is less affected (from ≈12.5±2.5 mM to ≈8.5±0.5 mM). This implies that the I G -to-B G transition is primarily controlled by NF-H subunit in ternary hydrogels. Thus, NF-M and NF-H sidearms in ternary NF hydrogels have distinct roles in controlling the salt concentrations at which the hydrogel transitions from the N G to I G and from the I G to B G phases, respectively. Both of these transitions involve large filament re-orientation (shown schematically in Fig. 3a ). Water retention capabilities of isotropic and LC hydrogels The macroscopic observations of differences in the hydrogel phases’ ability to maintain shape and volume hints at significant differences in their mechanical properties. 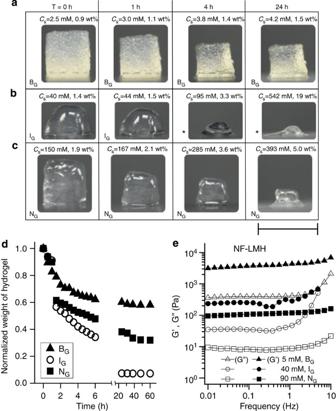Figure 4: Rheological and water retention behaviour. (a–c) Time-lapse photos of hydrogels in all three phases. Monovalent salt concentration and protein weight percentage for samples in each time frame are reported. Scale bar ≈5 mm. Bluish-opaque (BG) hydrogels (a) and to a lesser extent nematic (NG) hydrogels (c) have a remarkable ability to retain shape and volume, in stark contrast to isotropic (IG) hydrogels (b). Note that the BGhydrogel is whitish in appearance, due to the enhanced light scattering from the 5-mm thick gel, compared to the 1 mm bluish/partially opaque inFig. 2b,c. The asterisks that appear in (b)—at 4 and 24 h—indicate that samples that started in the IGphase atT=0 h show some birefringence at these later times (with much higher protein and salt concentrations). (d) Quantitative measurements of water retention as a function of time for the hydrogel samples in the BG, IGand NGphases (salt concentrations and protein wt% same as those in (a–c) forT=0). Remarkably BGand NGliquid-crystal hydrogels show plateau behaviour retaining ≈60 wt% and 30 wt% of their water over long times (up to 60 h of measurement time) with water loss occurring primarily during the first few hours. In contrast, isotropic hydrogels retains only 5 wt% of water after 24 h (also seeSupplementary Fig. S3andSupplementary Table S5). (e) Rheological measurements of elastic (G′) and viscous (G″) moduli of the hydrogels in the three phases. G′ and G″ are observed to decrease with increasing ionic strength indicative of the distinct electrostatic nature of the interfilament interactions in the three phases. All samples are equilibrated hydrogels of copolymer NF-LMH 44:31:25 wt% (≈7:3:2 mol ratio). In addition to the (1:1) salt concentration labelled in the figures, all samples included 1 mM MgCl2. Figure 4a–c shows such behaviour for the three phases in NF-LMH (7:3:2 mol ratio) hydrogels. The low C S B G hydrogel, cut as a cube, retains the sharp and irregular edges over time, and while the main volume reduction occurs in the first few hours, beyond that, there is very little change in volume between 4 h and 24 h (and over the few days of observation) ( Fig. 4a and Supplementary Fig. S3 ). In contrast, a clean straight edge does not form with the isotropic I G hydrogel, and any sharp edge tends to ‘round off’ as it is formed ( Fig. 4b and Supplementary Fig. S3 ). The highest salt concentration N G hydrogel has a smooth texture and tends to retain its shape after being cut into a cube; however, in contrast to B G hydrogels, it shrinks significantly between 4 h and 24 h ( Fig. 4c and Supplementary Fig. S3 ). Figure 4: Rheological and water retention behaviour. ( a – c ) Time-lapse photos of hydrogels in all three phases. Monovalent salt concentration and protein weight percentage for samples in each time frame are reported. Scale bar ≈5 mm. Bluish-opaque (B G ) hydrogels ( a ) and to a lesser extent nematic (N G ) hydrogels ( c ) have a remarkable ability to retain shape and volume, in stark contrast to isotropic (I G ) hydrogels ( b ). Note that the B G hydrogel is whitish in appearance, due to the enhanced light scattering from the 5-mm thick gel, compared to the 1 mm bluish/partially opaque in Fig. 2b,c . The asterisks that appear in ( b )—at 4 and 24 h—indicate that samples that started in the I G phase at T =0 h show some birefringence at these later times (with much higher protein and salt concentrations). ( d ) Quantitative measurements of water retention as a function of time for the hydrogel samples in the B G , I G and N G phases (salt concentrations and protein wt% same as those in ( a – c ) for T =0). Remarkably B G and N G liquid-crystal hydrogels show plateau behaviour retaining ≈60 wt% and 30 wt% of their water over long times (up to 60 h of measurement time) with water loss occurring primarily during the first few hours. In contrast, isotropic hydrogels retains only 5 wt% of water after 24 h (also see Supplementary Fig. S3 and Supplementary Table S5 ). ( e ) Rheological measurements of elastic (G′) and viscous (G″) moduli of the hydrogels in the three phases. G′ and G″ are observed to decrease with increasing ionic strength indicative of the distinct electrostatic nature of the interfilament interactions in the three phases. All samples are equilibrated hydrogels of copolymer NF-LMH 44:31:25 wt% (≈7:3:2 mol ratio). In addition to the (1:1) salt concentration labelled in the figures, all samples included 1 mM MgCl 2 . Full size image The changes in hydrogel volume were quantified by weight measurements of water loss with time ( Fig. 4d ). Consistent with the images in Fig. 4a , we see that the B G hydrogel loses water primarily during the first few hours and beyond 6 h retains ~60% of water over the 60 h of measurements. The I G hydrogel's water loss is quite rapid with ~7% water retention after 24 h. The N G phase shows behaviour similar to the B G , although with only 35% water retention over 60 h. This ability to retain shape and the largest amount of water over long times for the B G hydrogel is even more noteworthy as it contains the lowest protein fraction compared to the other two hydrogels (see protein concentrations in Fig. 4a–c (at time=0) and Supplementary Table S5 ). An important aspect of our finding, relating to the salt-responsiveness of the hydrogels, is that one may induce a transition from a water-retaining to a water-releasing hydrogel either by increasing C S (the B G -to-I G transition) or by decreasing C S (the N G -to-I G transition). NF hydrogel mechanical properties characterization To quantify the rheological properties of the gels, we measured the elastic (G′) and viscous (G″) moduli in ternary NF-LMH hydrogels (7:3:2 mol ratio) in the three different phases. As can be seen in Fig. 4e , the B G phase has a significantly larger elastic modulus (between a factor of 15 to 30) as compared to the I G and N G hydrogels, which have moduli comparable to other typical physical hydrogels [24] . The large value of G′, ranging between ≈3,000 and 7,000 Pa over a frequency range of 0.01–10 Hz, for the B G physical gel stabilized by electrostatic interactions at low C S (discussed in detail below), is comparable to the modulus of typical chemically crosslinked polyacrylamide hydrogels [25] . This enhanced mechanical property for the B G phase is consistent with its superior ability to retain shape and prevent water loss over long times. It is interesting to note that while the I G has a G′ modulus between the B G and the higher C S N G hydrogel, nevertheless, it loses water much more rapidly compared to either anisotropic LC hydrogel phase (B G or N G ). This implies that aside from the elastic modulus (which underlies the origin of prevention of water loss because of the necessary re-arrangement of the network upon volume reduction), the presence (B G , N G phases) or absence (I G phase) of orientational order is an important further factor in water retention. The microscopic structure data and mechanical behaviour of the three hydogels summarized in Figs 2 may be understood in the context of an electrostatic model of competing long-range interfilament repulsions and short-range sidearm attractions modulated by the buffer ionic strength. A recent electrostatic calculation based on the actual charge sequence of NF-L, NF-M and NF-H sidearms, with average phosphorylation, has shown that overlap configurations between oppositely charged anti-parallel sidearm residues on neighbouring filaments, may lead to energetically favourable short-range ionic attractions (see Supplementary Fig. S1 ) [23] . MD simulations of a (four-bead-reduced amino-acid) coarse-grained model of NF sidearms has also found attractive correlations between interpenetrating NF sidearms tethered to opposing planar surfaces [21] . The MD simulations are most relevant in the weak screening (that is, low salt concentration) regime. Thus, for the NF blue hydrogel (B G ) phase stable at low C S one expects that the polyampholyte nature of NFs will favour chain configurations where interpenetrating sidearms (from neighbouring filaments) form favourable cationic/anionic bonds (expanded view in Fig. 5a , depicting mostly zipped sidearms). 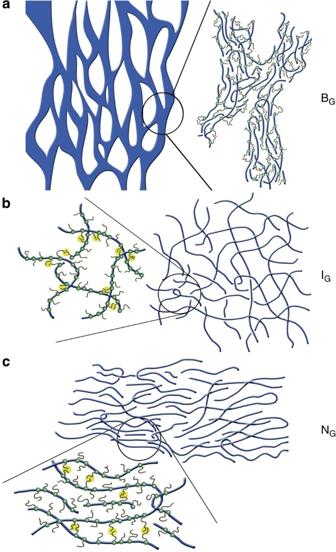Figure 5: Filament orientation and sidearm interactions. (a) At low salt concentration, the bluish-opaque (BG) liquid-crystal hydrogel exhibits microphase separation of high and low NF protein concentration domains, as discussed in the text. The expanded view, with on-average parallel filament orientation but heterogeneity (that is, distribution) in interfilament spacing, shows short-range sidearm attractions between anionic/cationic residues (that is, ‘zipped’ sections) consistent with recent electrostatic calculations23and MD simulations21showing energetically favourable configurations for sidearm attractions (see alsoSupplementary Fig. S1). (b) At intermediate salt concentrations, partial unzipping of sidearms leads to random crossed-filament orientation in the isotropic gel (IG) phase, which lowers the longer-ranged electrostatic repulsion between filaments due to their net-negative sidearms. (c) At high salt concentrations, screening of the interfilament electrostatic repulsions leads to an Onsager-like nematic hydrogel (NG) with parallel filament orientation. The yellow highlights in (b) and (c) denote transient (weaker) electrostatic attractions between some fraction of sidearms in the IGand NGphases. In contrast, in the low salt concentration (bluish-opaque gel (BG)) phase (a) the sidearm interactions are stronger and less transient. Figure 5: Filament orientation and sidearm interactions. ( a ) At low salt concentration, the bluish-opaque (B G ) liquid-crystal hydrogel exhibits microphase separation of high and low NF protein concentration domains, as discussed in the text. The expanded view, with on-average parallel filament orientation but heterogeneity (that is, distribution) in interfilament spacing, shows short-range sidearm attractions between anionic/cationic residues (that is, ‘zipped’ sections) consistent with recent electrostatic calculations [23] and MD simulations [21] showing energetically favourable configurations for sidearm attractions (see also Supplementary Fig. S1 ). ( b ) At intermediate salt concentrations, partial unzipping of sidearms leads to random crossed-filament orientation in the isotropic gel (I G ) phase, which lowers the longer-ranged electrostatic repulsion between filaments due to their net-negative sidearms. ( c ) At high salt concentrations, screening of the interfilament electrostatic repulsions leads to an Onsager-like nematic hydrogel (N G ) with parallel filament orientation. The yellow highlights in ( b ) and ( c ) denote transient (weaker) electrostatic attractions between some fraction of sidearms in the I G and N G phases. In contrast, in the low salt concentration (bluish-opaque gel (B G )) phase ( a ) the sidearm interactions are stronger and less transient. Full size image The B G hydrogel phase is stable for C S less than ≈10 mM salt ( λ D =Debye length≥30 Å; λ D =3.04/( M ) 0.5 Å for 1:1 electrolytes, with M being the salt molarity) for NF-LH and NF-LMH and less than ≈40 mM salt ( λ D 15 Å) for NF-LM hydrogels, respectively. Thus, within our model, the B G hydrogel is stable in the regime where the Debye length is comparable to or larger than the ‘single-chain’ NF sidearm persistence length, and hence the regime where large regions of the unstructured segments of opposing chains are electrostatically correlated (the NF sidearm persistence length, l p , is expected to be comparable to that of unstructured single-stranded RNA (with l p between 11 Å and 30 Å (ref. 26 )), which has a similar net negative charge per unit length.). In this regime, strong electrostatic attractions between oppositely charged residues, on opposing sidearms less than λ D apart, will potentially lead to many zipped regions. In addition to the electrostatic contributions considered in previous calculations [21] , [23] , the release of counter-ions (present near the charged residues of the sidearms due to Manning condensation at low salt concentrations [27] ), upon ionic bond formation, is an additional entropic driving force ‘zipping’ sidearms [28] , [29] , [30] . On the larger micron-length scale the partial bluish-opaque colour and enhanced SAXS suggest a spatially heterogeneous microstructure [31] , with the B G phase consisting of a microphase-separated hydrogel where interconnected regions of high protein density—with net-negative finite-sized aligned NF bundles—are separated by hydrated pockets with released counter-ions ( Fig. 5a ). We point out that thicker samples of B G hydrogels with enhanced light scattering are white in appearance (compare 5 mm samples in Fig. 4a to 1 mm samples in Fig. 2b,c ). This microphase-separated model of the B G phase (that is, a network of aligned NF bundles) is consistent with the SAXS correlation peaks, which shows that the spatially heterogeneous B G hydrogel and the optically transparent spatially homogeneous N G hydrogel have comparable average interfilament spacings ( Fig. 3 ) even though the B G hydrogel is a more dilute hydrogel with nearly half the volume fraction of protein (see Supplementary Tables S1–S4 ). With increasing C S , the anionic/cationic electrostatic bonds are weakened in the B G hydrogel where increased screening begins to partially ‘unzip’ the sidearms, thus, melting away much of the short-range attractions. The system then transitions to the optically transparent isotropic I G hydrogel with randomly oriented NF filaments crossing at large angles ( Fig. 5b ). In this regime of intermediate screening (sandwiched between the low (B G ) and high (N G ) screened phases), the longer-ranged repulsive forces, due to the large net negative charge of the filament sidearms, drives the random crossed-filament geometry of the I G phase, which is energetically favored over the parallel orientation of the B G phase [32] . Indeed, crossed-filament orientations have previously been reported for filamentous actin, a highly net negative-charged cytoskeletal filament, at low salt concentrations [33] , [34] . At even higher C S , the longer-ranged repulsive forces are increasingly more screened, and at some critical salt concentration lead to the transition from the I G phase to the optically transparent and birefringent nematic N G hydrogel with aligned filaments ( Fig. 5c ). This transition into the nematic hydrogel phase arises from an effective Onsager ordering; that is, upon screening of the longer-ranged electrostatic repulsions, the overall gain in translational entropy is larger than the loss of orientational entropy for semiflexible filaments when the ratio of the persistence length (for l p <contour length) to the filament width is >5.1 (refs 35 , 36 ). For reconstituted NFs with a persistence length l p between ≈100 and 150 nm (ref. 37 ) (comparable to the contour length ≈200 nm) and filament diameter D≈10 nm, l p /D≈10–15. Thus, one expects the I G hydrogel to transition to the nematic N G phase when electrostatic interactions are screened. The microscopic structure of the B G hydrogel, with ‘multiple cationic/anionic junction zones’ within the finite-sized NF bundles (expanded view, Fig. 5a ), naturally leads to a hydrogel network with a large amount of ionic linking relative to the linking due to the weaker transient ionic sidearm interactions in the I G and N G hydrogels at higher C S (expanded views in Fig. 5b,c ). This is consistent with the enhanced elastic modulus in the B G hydrogel phase. An interesting observation is that although I G and N G hydrogels show high stickiness to the glass substrate, B G hydrogels lack any stickiness to hydrophilic surfaces and readily slide as a solid body when pushed on glass. This is again consistent with the microscopic picture of the B G hydrogel with a large fraction of zipped cationic/anionic bonds (that is, unzipped charged residues are a source of stickiness). In summary, we have described the existence of three sidearm-mediated hydrogel phases with decreasing ionic strength with an isotropic (I G ) phase with crossed-filament orientation sandwiched between two parallel filament hydrogel phases (N G and B G ). NF-LH networks stabilize the isotropic hydrogel over a wide salt concentration range whereas NF-LL and NF-LM networks favour the nematic N G hydrogel over a wide salt concentration range (except for a very narrow C S region for NF-M where the crossed orientation is favored). Comparing the sidearm charge distribution patterns ( Fig. 1c and Supplementary Fig. S1 ) one sees that all three contain large blocks of net-negative domains with interspersed and flanking cationic residues (residues ~446–547 for NF-L, ~452–848 for NF-M and ~412– 789 for NF-H). A notable difference is the additional long stretch of randomly distributed cationic/anionic charge residues—with a nearly net zero charge—in NF-H from the middle of the sidearm to the C-terminus (residues 790–1090, net charge≈−6e). Such an ampholytic section is not present in NF-L and present only as a much shorter segment at the C-terminus for NF-M (residues 849–926). This suggests that this very weakly charged (and thus more flexible) polyampholyte section in the NF-H sidearm has an important role in stabilizing the I G hydrogel with random, crossed filaments (that is, orientational flexibility) at intermediate salt concentrations. On the other hand, the NF-M and NF-L sidearms, which are dominated by the large net-negative blocks with interspersed and flanking cationic domains, favour LC hydrogels with parallel filament orientation. We point out that the smaller net negative charge of the NF-L sidearms (≈−40e) compared to that for phosphorylated NF-M (≈−90e) and NF-H (≈−92e), leading to a smaller electrostatic interfilament repulsion, may be a further contributing factor to the lack of the isotropic I G phase for NF-LL hydrogels. Future MD simulations of NF sidearm interactions as a function of varying ionic strength, taking into account the actual net charge and charge pattern in the sidearms [21] , [38] , is much needed to look for direct correlations between sidearm charge distribution pattern and the relative preference for the crossed versus parallel filaments orientations. Our results show that filament re-orientation flexibility of the NF network, in the physiologically relevant N G phase, requires NF-LH with ≈70:30 wt% subunit composition, with little or no NF-M subunits, in order to ensure that the N G –I G transition (that is, where the parallel to crossed-filament re-orientation is facilitated) occurs close to physiological salt concentrations ≈85 mM KCl. In axons the local phosphorylation state of the sidearm together with the salt concentration will determine the relative stability of the parallel versus crossed-filament orientation state of the network. This suggests that facilitated axonal transport (that is, where organelles larger than the NF network mesh size are transported along microtubules immersed in the network) would require the presence of subunit composition variations along the cross-section of axons, with NF-LH-dominant regions in the vicinity of microtubule tracks, to ensure optimal NF filament re-orientation flexibility. In addition to the biological interest in NFs as a critical component of the cytoskeleton, the NF hydrogels are also interesting from the biomaterials perspective. Environmentally responsive polymers and hydrogels have been the inspiration of multiple studies [39] , [40] . The reversible tunability of the hydrogel elastic modulus, switching between a high modulus B G phase (comparable to a crosslinked chemical hydrogel) and much lower moduli I G and N G phases (comparable to physical gels), in response to changes in ionic strength, is a significant new property of these polyampholyte-based salt-responsive hydrogels distinguishing them from irreversibly crosslinked gels. More broadly, the findings reported here pave the way for a new approach utilizing ‘polyampholyte’ linking elements in developing biomimetic versions of the natural NF hydrogels with rapid and reversible cycling between high and low elastic moduli and structure-dependent water retention and release properties. Purification Bovine spinal cords were kept on ice until the time of preparation (several hours later). The bovine spines were homogenized in equal parts of buffer A (100 mM MES buffer, 1 mM MgCl 2 , 1 mM EGTA, 0.1% sodium azide, adjusted to pH 6.8 by adding ≈85 mM NaOH), and then clarified of cellular debris by centrifugation, with the NFs persisting in the supernatant. Successive steps of solution centrifugation, which include a 50% glycerol NF-enriched solution in buffer A followed by NF solution layering on a sucrose gradient (0.8 M sucrose on 1.5 M sucrose in buffer A), were performed to further enrich the solution of NFs and remove contaminating proteins while not disrupting single-filament integrity. The outcome of these steps, collectively referred to as the crude purification [22] , [23] , [41] , is the native ternary NF-hydrogel, contaminated with co-sedimenting proteins. The crude fraction is then denatured using 8 M urea, where anion exchange column chromatography enables the separation of all three subunits from one another and from all contaminating proteins. The denatured crude fraction is first applied to a DEAE–cellulose (Sigma Aldrich, St Louis, MO) resin, where various buffer elutions produce two fractions: the first, eluted using buffer B (0.1 M sodium phosphate and 0.1 vol% 2-mercaptoethanol in 8 M urea, pH=6.5), is enriched in NF-H and the majority of the contaminating proteins; and the second, eluted using buffer B with 55 mM NaCl at pH=7.0, is mainly enriched in NF-L and NF-M. These two fractions are exclusively added to a hydroxylapatite resin (Bio-Gel HT gel, Bio-Rad, Hercules, CA, USA), producing pure fractions of each of the subunits. Fractions were concentrated using Centricon tubes (Millipore, Billerica, MA, USA) and their purity checked with 7.5% SDS–PAGE (see Supplementary Fig. S4 ). Sample protein concentrations were determined using the Bradford assay. Upon reconstitution from purified subunits, single-filament AFM studies [37] show that the 10 nm reconstituted NF filaments exhibit the characteristic repeated bead-like structure of native 10 nm NFs [10] . Typical AFM images of our preparations adapted from ref. 23 are shown in Supplementary Fig. S4 . The main difference between native NFs (with contour length on the order of a few microns [10] ) and reconstituted NFs is that the latter have a shorter contour length of ≈200 nm (ref. 37 ). Thus, although the single-molecule properties between NFs with small and long contour lengths will be different, we expect that the shorter contour length should not lead to significantly different properties (both microscopic and macroscopic) of the extended NF network hydrogels compared to networks consisting of longer native filaments. First, the 22-nm lateral distance between C-terminal sidearms, which is about a tenth of the contour length of reconstituted NFs, allows for a large number of interfilament links (that is, due to interactions between C-terminal sidearms) per reconstituted NF. Second, our SAXS data show that the interfilament spacings for NF-LM and NF-LMH hydrogels ( Fig. 3b,d ) closely match spacings obtained by cryo-TEM studies of the native NF networks in dendrites (consisting of NF-LM [42] ) and axons (consisting of NF-LMH [43] ), respectively. Thus, we expect the mesh size to be similar for networks comprising either wild-type NFs or reconstituted NFs. Taken together, we expect both microscopic and macroscopic properties to be nearly the same in reconstituted and native NF networks. Hydrogel formation The subunits (NF-L, NF-M and NF-H), still in urea, are recombined in desired ratios, and set to dialyse against buffer A for 24 h, which allows for filament assembly. The buffer is then exchanged to 40 mM MES buffer A (which includes ≈30 mM of NaOH to achieve pH=6.8), and left to dialyse for another 12 h. For protein samples with the desired (1:1) salt concentration less than the NaOH ion concentration present in the 40 mM MES buffer A (≈30 mM), the solutions are diluted with milliQ; conversely, for samples with a desired salt concentration higher than ≈30 mM NaOH, a stock of KCl solution was used to increase the sample salt content. The divalent concentration was fixed at 1 mM MgCl 2 for all samples. Post-dialysis protein solutions are diluted to 4 mg ml −1 and sedimented at 100,000 g for 1 h at room temperature. Post-centrifugation, the excess solvent is removed and exchanged with an excess of the desired buffer, and the gels are allowed to equilibrate (swell). The remnant solvent is again removed. All chemicals were from Sigma Aldrich and used without further purification. Salt buffer preparation A stock of buffer C (buffer A lacking sodium azide) is used to make the subsequent buffers (only used post purification) with variable monovalent salt concentrations. The salinity of the buffer was adjusted using different amounts of NaOH (needed to ensure a constant pH of 6.8) and KCl. Lower MES buffer concentrations were used to make the low-salt buffers (as less NaOH would be needed to achieve the desired pH). The MgCl 2 concentration was fixed at 1 mM (as well as EGTA at 1 mM). Capillary sample preparation The post-dialysis protein solution is aliquoted to ensure 150 μg of NF protein per capillary sample, and spun down using Beckman Airfuge (Rotor A-10/30). The resultant equilibrated hydrogels are transferred to 1.5 mm quartz capillaries (Hilgenberg, GmBh), sedimented at low speeds, followed by the addition of excess desired buffer and the capillaries are then flame-sealed. Polarized optical microscopy and SAXS experiments The capillary samples are observed using a Nikon 282130 microscope fitted with a × 5 objective, and imaged with a Nikon Coolpix P5000 camera fitted with a MDC lens. SAXS experiments were conducted on the equilibrated hydrogel samples (in the same quartz capillaries) at the Stanford Synchrotron Radiation Laboratory (SSRL BL4-2), acquired on a MarCCD 165 (Fiber Optic-Taper coupled CCD) detector. Scattering data were collected using X-rays with wavelength 1.3776 Å and a sample-to-detector distance of ≈3.5 m. The unoriented data was integrated over 360° using ‘Nika’ for Igor Pro [44] to yield the scattering profile. Test samples determined optimal exposure time, and the experimental samples were run for half the exposure time where radiation damage was first observed. An arbitrary background (set as an exponential decay of intensity versus q -value) was subtracted from the individual scattering profiles and fit to Gaussians to determine peak positions. The same profiles were also fit in an alternate manner, as a verification: backgrounds in the form of a linear line in log–log plots were subtracted from the profiles, which were then fit to Lorenzian functions. Both methods yielded comparable peak values, to within ±2%. Monitoring hydrogel phase reversibility To achieve the new desired monovalent salt concentrations, calculated volumes of stock KCl and stock MgCl 2 solutions and milliQ water were added to the buffer solution immersing the pre-equilibrated hydrogels in unsealed quartz capillaries. Immediately after, the new buffer mixture is exchanged with a fresh aliquot of the desired buffer. Simultaneous to buffer exchange, the hydrogels were imaged using the polarized optical microscope (see above) to elucidate the reversibility routes between the three phases, and monitor their rates where allowed. While the reversibility experiments as described gave consistent results, one experiment from one particular protein batch (out of >10 batches that were purified in this study), showed a gel-to-sol transition in lowering the salt concentration from a relatively high-salt N G hydrogel state of ≈240 mM to an intermediate-salt I G phase (with a one-step buffer removal followed by new buffer addition). Time-lapse imaging and drying experiment Equilibrated hydrogels are shaped, then placed on a clean glass slide, and imaged using a Nikon D300 camera mounted on a tripod (Lens: Nikon 50 mm f/1.8D AF Nikkor Lens attached to a Vivitar × 2 macro focusing teleconverter), with the lens set at maximal exposure. Identical hydrogels are mounted onto separate clean glass slides, and weighed at select time-intervals. Hydrogels in each of the three phases were also retained in their ultracentrifuge tubes post-centrifugation and equilibration, to normalize over surface area, and also weighed at select time-intervals. This demonstrated that the drying profiles were due to the intrinsic properties of the gel, rather than gel shape (see Supplementary Fig. S3 ). Rheology Large volume samples were ultracentrifuged to form larger hydrogels necessary for the rheological measurements. An agarose gel ‘stopper’ was polymerized at the bottom of the ultracentrifuge tubes before layering the NF solution to ensure the formation of a uniform and shape-reproducible disk-like sample. The viscoelastic response of equilibrated NF hydrogels is determined by measuring the frequency-dependent storage modulus G′ ( ω ) and loss modulus G″ ( ω ) with a stress-controlled rheometer (Physica MCR 301; Anton Paar) over a frequency range of three decades. Gels are preformed into an appropriate shape and carefully loaded into the rheometer. Measurements are conducted at 21 °C using an 8-mm plate–plate geometry. Plate separation was adjusted to match the samples geometry. To ensure a linear response, small torques (≈0.5 μNm) are applied. A solvent trap is placed around the sample to prevent the artifacts from drying. How to cite this article: Deek, J. et al. Neurofilament sidearms modulate parallel and crossed-filament orientations inducing nematic to isotropic and re-entrant birefringent hydrogels. Nat. Commun. 4:2224 doi: 10.1038/ncomms3224 (2013).